Trunk exoskeleton in teleosts is mesodermal in origin The vertebrate mineralized skeleton is known to have first emerged as an exoskeleton that extensively covered the fossil jawless fish. The evolutionary origin of this exoskeleton has long been attributed to the emergence of the neural crest, but experimental evaluation for this is still poor. Here we determine the embryonic origin of scales and fin rays of medaka (teleost trunk exoskeletons) by applying long-term cell labelling methods, and demonstrate that both tissues are mesodermal in origin. Neural crest cells, however, fail to contribute to these tissues. This result suggests that the trunk neural crest has no skeletogenic capability in fish, instead highlighting the dominant role of the mesoderm in the evolution of the trunk skeleton. This further implies that the role of the neural crest in skeletogenesis has been predominant in the cephalic region from the early stage of vertebrate evolution. The mineralized skeleton is one of the major innovations of vertebrates, assuring active locomotion and better protection for survival. It is thought to have emerged initially as exoskeletonal elements because early fossil fish such as ostracoderms (armored fish) were extensively covered by dermal bone and dentine yet lacked a mineralized endoskeleton [1] , [2] . The exoskeleton is retained in the form of dermal dentine scales in cartilaginous fish and dermal scales and fin rays in bony fish. During terrestrial evolution, however, it has been drastically reduced or lost in the trunk region, and the mesoderm-derived endoskeleton (vertebra) has become the major source of structural support [3] , [4] ( Fig. 1 ). The emergence of the neural crest, an embryonic tissue, in early vertebrates is known to be closely related to the novel characteristics unique to vertebrates [5] . Indeed, most of the cranial exoskeletal elements in tetrapods such as teeth and dermal skull roof are derived from the neural crest [6] , [7] , [8] , [9] , [10] , [11] . However, the embryonic origin of the trunk exoskeleton remains largely unknown and thus the role of the neural crest in the early evolution of vertebrate skeletal system is still unclear. 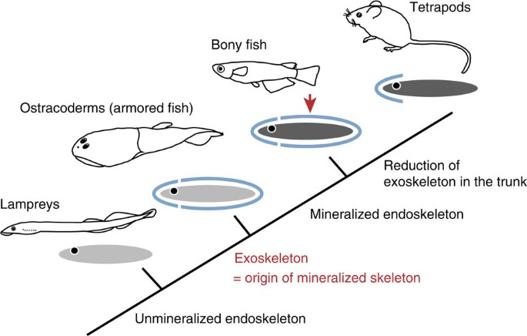Figure 1: Origin and evolution of mineralized skeleton in vertebrates. Vertebrates have two distinct sets of skeletons, exoskeleton (dermal skull roofs, teeth, scales, fin rays and so on.) and endoskeleton (neurocranium, vertebra, appendicular skeleton and so on). While the endoskeleton consists of endochondral bones that are preformed by cartilage and later replaced by mineralized bones, the major components of the exoskeleton are the dermal bones that develop in the dermis only by membranous ossification. A mineralized skeleton is thought to have emerged initially as exoskeletonal elements. Bony fish retain the exoskeleton in the form of dermal scales and fin rays. During terrestrial evolution, however, the exoskeleton has been drastically reduced or lost in the trunk region. Outer blue circles show the exoskeleton. Inner solid pale circles show the unmineralized endoskeleton. Inner solid-dark circles show the mineralized endoskeleton. The red arrow indicates the trunk exoskeleton we focused on in the present experiment. Figure 1: Origin and evolution of mineralized skeleton in vertebrates. Vertebrates have two distinct sets of skeletons, exoskeleton (dermal skull roofs, teeth, scales, fin rays and so on.) and endoskeleton (neurocranium, vertebra, appendicular skeleton and so on). While the endoskeleton consists of endochondral bones that are preformed by cartilage and later replaced by mineralized bones, the major components of the exoskeleton are the dermal bones that develop in the dermis only by membranous ossification. A mineralized skeleton is thought to have emerged initially as exoskeletonal elements. Bony fish retain the exoskeleton in the form of dermal scales and fin rays. During terrestrial evolution, however, the exoskeleton has been drastically reduced or lost in the trunk region. Outer blue circles show the exoskeleton. Inner solid pale circles show the unmineralized endoskeleton. Inner solid-dark circles show the mineralized endoskeleton. The red arrow indicates the trunk exoskeleton we focused on in the present experiment. Full size image Teleost scales (elasmoid scales) have recently been re-evaluated as odontogenic exoskeletal structures, like teeth, because of their development and structure [12] , [13] . During scale development, a papilla is formed in the dermis immediately adjacent to the basal layer of the epidermis, followed by differentiation of enamel-like capping tissue, a type of dentin (external layer) and a plywood-like tissue (elasmodin). These tissues are comparable with those of odontogenic components of ancestral rhombic scales [12] , [13] . Fin rays are also considered to be derivatives of the ancestral scales [14] , [15] . Therefore, elucidating the embryonic origin of these trunk exoskeletal elements could provide critical implications for understanding the evolution of mineralized skeletons. Previously, the contribution of the neural crest to the formation of scales and fin rays has been suspected by the observations that goldfish tumour pigment cells were able to transform into scales in vitro [16] , and that labelled neural crest cells exhibited invasive behaviour into fins in zebrafish and swordtail [17] , [18] . However, these cells had not been traced for an extended period of time to analyse their contribution to exoskeletal elements mainly due to technical difficulties in long-term cell-lineage analysis in fish. In this study, we have applied recently developed long-term labelling methods to medaka fish. The first method was transplantation of labelled tissues, using a modified zebrafish protocol [19] , [20] ( Fig. 2 ). In this method, we used double transgenic medaka as donors, β-actin-DsRed / osterix-EGFP . This transgenic fish enabled us to track the DsRed-positive transplanted donor cells throughout development under the ubiquitous β-actin promoter, and simultaneously to judge if these cells differentiated into bone-forming cells (odontoblasts/osteoblasts) by detecting osterix driven green fluorescent protein (GFP) expression ( Fig. 2 , Supplementary Fig. S1 ) ( osterix is a transcription factor whose expression marks the intermediate stage in bone-forming cell differentiation [21] , [22] ). The main results obtained were then confirmed by the second long-term labelling technique using the infrared laser-evoked gene operator (IR-LEGO) system (Fig. 4a) (refs 23 , 24 ). By these methods, we found that bone-forming cells in both scales and fin rays are derived from the mesoderm, not the neural crest, suggesting that the trunk neural crest has no skeletogenic capability in fish. 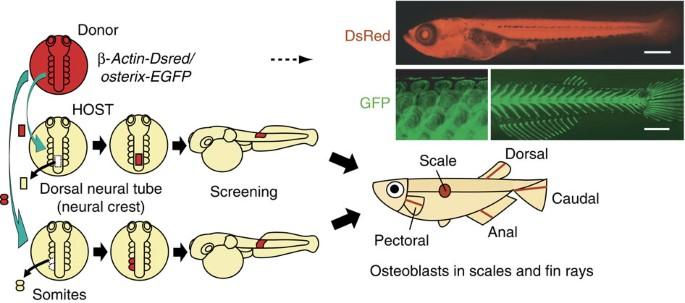Figure 2: The scheme of the transplantation experiments. We replaced dorsal neural tubes (including neural crest cells) or somites of host embryos with transgenic donor ones at the 12- to 30-somite stages. After screening for successful transplants at the hatching stage, we examined the contribution of neural crest cells and somite cells to scales and fin rays. The insets show the donor fish ubiquitously expressing DsRed (upper, 3 days post hatching; 3 dph) and odontoblast/osteoblast-specific GFP in scales (lower left, 3-week post hatching; 3 wph) and fin rays (lower right, 2 wph). Scale bars, 200 μm. Figure 2: The scheme of the transplantation experiments. We replaced dorsal neural tubes (including neural crest cells) or somites of host embryos with transgenic donor ones at the 12- to 30-somite stages. After screening for successful transplants at the hatching stage, we examined the contribution of neural crest cells and somite cells to scales and fin rays. The insets show the donor fish ubiquitously expressing DsRed (upper, 3 days post hatching; 3 dph) and odontoblast/osteoblast-specific GFP in scales (lower left, 3-week post hatching; 3 wph) and fin rays (lower right, 2 wph). Scale bars, 200 μm. Full size image Scales and median fin rays are derived from the somite We first examined the contribution of neural crest cells to scales and median fin rays by replacing dorsal neural tubes (including neural crest cells) of host embryos with transgenic donor ones at the 12- to 30-somite stages at the level of newly formed somites. As a transgenic line expressing a reporter gene in neural crest cells is not available in medaka, we confirmed a successful transplantation of neural crest cells by the following two methods. First, a genetic marker of pigmentation was used; we had introduced the black melanophore gene ( B/B ) into the donor strain while the hosts had the colourless allele ( b/b ) ( Supplementary Fig. S1 ). We observed melanophores in transplanted host embryos and juvenile fish ( Fig. 3e ). Second, we performed a histological examination of transplanted host embryos stained with anti-DsRed antibody. As shown in Fig. 3a , DsRed-positive donor cells exhibit the typical shape and position of migrating neural crest cells, as well as dorsal neural tube cells, confirming that only neural tubes with neural crest cells were transplanted. 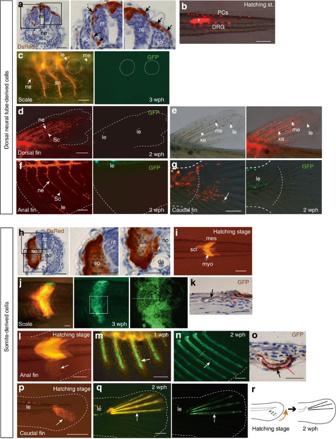Figure 3: Somite origin of scales and median fin rays revealed by tissue transplantation. (a,h) Cross-sections of the host embryos 12 h after transplantation (after healing of skin wounds) of dorsal neural tubes and somites at 18-somite level, respectively. DsRed detection was performed by immunostaining. Arrows likely show migrating neural crest cells. (b,i) Screening for successful transplants at hatching stage after transplantation of dorsal neural tube and somite, respectively. An asterisk shows neural tube. (c,d,f,g) DsRed (left) and GFP (right) images of dorsal neural tube-derived cells in the trunk surface (c), dorsal (d), anal (f) and caudal fins (g). Dotted circles incindicate scales. (e) A bright-field (left) and merged images with DsRed (right) in the region shown ind, showing that most of the DsRed-positive cells are pigment cells. (j) Orange: DsRed-positive somite-derived cells in the trunk surface (the fluorescence is mostly from the muscle). Green and yellow: GFP-positive bone-forming cells in scales. Right, the enlarged image of the region shown as the box in the middle panel. (l,p) Invasion of mesenchymal cells into the anal and caudal fin primordia. (m,n,q) Orange: DsRed-positive somite-derived cells in the anal (m) and caudal (q) fins. Green: GFP-positive bone-forming cells. (k,o) Histological sections at the level of dotted lines inj(right) andn, respectively. Black and red arrows show bone-forming cells and bone matrix, respectively. (r) Caudal fins bend dorsally during larval stages. All the live images are lateral views. Anterior to the left. Emission filters: DsRed (590–650 nm) forb,d(left),e(right),f(left),g(left),i,l,p; GFP2 (or long path filter, >510 nm) forc(left),j(left),m,q; GFP3 (500–550 nm) for the panels on the right ofc,d,f,g,j,n,q, and the middle panel ofj. da, dorsal aorta; DRG, dorsal root ganglia; le, leucophore (autofluorescent); me, melanophore; mes, mesenchyme; myo, myotome; ne, neuron; nt, neural tube; no, notochord; PCs, pigment cells; Sc, Schwann cell; scl, sclerotome; sn, spinal nerve; so, somite; xa, xanthophore. Scale bars, 50 μm (a,h,k,o), 500 μm (b–g,i,j,l–n,p,q). Figure 3: Somite origin of scales and median fin rays revealed by tissue transplantation. ( a , h ) Cross-sections of the host embryos 12 h after transplantation (after healing of skin wounds) of dorsal neural tubes and somites at 18-somite level, respectively. DsRed detection was performed by immunostaining. Arrows likely show migrating neural crest cells. ( b , i ) Screening for successful transplants at hatching stage after transplantation of dorsal neural tube and somite, respectively. An asterisk shows neural tube. ( c , d , f , g ) DsRed (left) and GFP (right) images of dorsal neural tube-derived cells in the trunk surface ( c ), dorsal ( d ), anal ( f ) and caudal fins ( g ). Dotted circles in c indicate scales. ( e ) A bright-field (left) and merged images with DsRed (right) in the region shown in d , showing that most of the DsRed-positive cells are pigment cells. ( j ) Orange: DsRed-positive somite-derived cells in the trunk surface (the fluorescence is mostly from the muscle). Green and yellow: GFP-positive bone-forming cells in scales. Right, the enlarged image of the region shown as the box in the middle panel. ( l , p ) Invasion of mesenchymal cells into the anal and caudal fin primordia. ( m , n , q ) Orange: DsRed-positive somite-derived cells in the anal ( m ) and caudal ( q ) fins. Green: GFP-positive bone-forming cells. ( k , o ) Histological sections at the level of dotted lines in j (right) and n , respectively. Black and red arrows show bone-forming cells and bone matrix, respectively. ( r ) Caudal fins bend dorsally during larval stages. All the live images are lateral views. Anterior to the left. Emission filters: DsRed (590–650 nm) for b , d (left), e (right), f (left), g (left), i , l , p ; GFP2 (or long path filter, >510 nm) for c (left), j (left), m , q ; GFP3 (500–550 nm) for the panels on the right of c , d , f , g , j , n , q , and the middle panel of j . da, dorsal aorta; DRG, dorsal root ganglia; le, leucophore (autofluorescent); me, melanophore; mes, mesenchyme; myo, myotome; ne, neuron; nt, neural tube; no, notochord; PCs, pigment cells; Sc, Schwann cell; scl, sclerotome; sn, spinal nerve; so, somite; xa, xanthophore. Scale bars, 50 μm ( a , h , k , o ), 500 μm ( b – g , i , j , l – n , p , q ). Full size image At the hatching stage, the successful transplants that properly exhibited DsRed-positive dorsal root ganglia and pigment cells, major neural crest derivatives in the trunk region, were screened ( Fig. 3b ) and then raised until 2–3 weeks of age when each organ fully developed ( Fig. 2 ). These larvae contained a significant number of DsRed-positive cells in the trunk surface, irrespective of the level of transplantation (that is, 12- to 30-somite levels) ( Fig. 3c ), and DsRed-positive cells were also seen in the developing median fins when transplanted at the 17- to 20-somite levels for dorsal fins, 12- to 18-somite levels for anal fins, and 24- to 30-somite levels for caudal fins ( Fig. 3d , left). However, in both trunk and fins, we did not detect any GFP signal driven by the osterix promoter, indicating that neural crest-derived cells do not differentiate into bone-forming cells in the dermis and median fins ( n =0/38, 0/19, 0/15, 0/13 for scales, dorsal, anal and caudal fins, respectively; for scales, number of fish with GFP signals in scales/number of fish of successful transplantation judged at the hatching stage; for fins, number of fish with GFP signals in fins/number of fish having DsRed-positive cells in their fins at later stages) ( Fig. 3c , right). From colour and morphology, dorsal neural tube-derived cells are likely to include pigment cells, peripheral neurons and Schwann cells ( Fig. 3c ). To exclude the possibility that some populations of neural crest cells that would contribute to bone-forming cells had already migrated out from the dorsal neural tube of donor embryos at the time of operation, we checked the expression of foxd3 , a pan-neural-crest marker, in both whole donor embryos and isolated neural tubes that are to be transplanted. We confirmed that no signal for foxd3 could be seen outside the neural tube and that foxd3 -expressing cells still remained on the dorsal neural tube in vivo and isolated ones as well, indicating that an intact neural crest cell population was replaced at the level of transplantation ( Supplementary Fig. S2 ). We also confirmed that the neural crest does not contribute to trunk endoskeleton such as vertebrae and fin radials (data not shown). We then asked which lineage of cells contributes to scales and fin rays instead of neural crest cells. We considered the derivatives of the somite as alternative candidates because somite-derived cells are known to constitute the dermis of zebrafish [25] and median fin mesenchyme in axolotl [26] , catshark [27] and zebrafish [25] . However, in those studies cells were not traced until the stage when bone-forming cells differentiate in scales and fin rays. Thus, we transplanted somites from the transgenic donor embryos into non-transgenic hosts at nearly the same stages and the same anteroposterior (AP) levels as performed in the above neural tube transplantation. Histological sections of the transplants again confirmed the accuracy of somite transplantation; only somite cells were labelled ( Fig. 3h ). Like the neural tube transplantation experiment, successful transplants with DsRed-positive myotome, sclerotome and mesenchyme were screened at the hatching stage ( Fig. 3i ), and grown for 2–3 weeks. We found that the DsRed-positive cells colonized on scales and expressed GFP, indicating that they differentiated into bone-forming cells ( n =39/39, Fig. 3j ). GFP-positive scales were found at nearly all dorsoventral levels, overlying the DsRed-expressing myotome ( Fig. 3j , left). Similarly, in each host median fin, DsRed-positive cells invaded into young fin folds yet to develop fin rays ( Fig. 3l , Supplementary Fig. S3a ) and began to express GFP ( Fig. 3m , Supplementary Fig. S3b ) when transplanted 17- to 20-somite for dorsal fins, 12- to 18-somite for anal fins, and 26- to 30-somite for caudal fins. GFP expression persisted as the fish grew and eventually was seen in entire fin rays ( n =14/16, 11/11, and 11/12 for dorsal, anal, and caudal fins, respectively) ( Fig. 3n , Supplementary Fig. S3c ). In histological sections, GFP-positive cells exhibit the typical shape of bone-forming cells in scales and fin rays in close contact with the bone matrix, confirming that they are indeed odontoblasts/osteoblasts (black arrows in Fig. 3k ). To control for the contamination of neural crest cells, we again used the genetic marker for pigmentation; donor tissues were derived from wild-type ( B/B ), while the hosts had the colourless allele ( b/b ) ( Supplementary Fig. S1k,l ). We never obtained transplants with black melanophores ( n =135), indicating that neural crest cells (at least melanophore-producing crest cells) were not carried over during transplantation. Labelling of somite cells by IR-LEGO To further confirm the somite origin of scales and median fin rays, we adopted the second long-term labelling method, IR-LEGO, which can induce the heat-shock response in target cells upon irradiation with an infrared laser [23] , [24] , in combination with cre-loxP [28] . A newly formed somite of double transgenic embryos obtained from the cross between hsp-cre and β-actin -loxP[ DsRed ]- EGFP was exposed to infrared laser from the dorsal side at the same stages and the same AP levels as performed in the somite-transplantation experiment ( Fig. 4a ). We targeted cells at the lateral side because they are known to give rise to dermis and dorsal fin cells in zebrafish [25] . Within 12 h after irradiation, a small population of cells (~5–10 cells) was irreversibly labelled with GFP and thus could be tracked for life ( Fig. 4b , Supplementary Fig. S4 ). We used a low laser intensity so as to theoretically target a single cell [23] , but we were unable to precisely determine the number of irradiated cells because it took at least 12 h for cells to express mature GFP, during which cell divisions may have taken place. Three days after irradiation (st.35, 5 dpf), some GFP-positive cells invaded into growing fin folds while most of the labelled cells contributed muscle cells (data not shown). Three to four weeks after irradiation, GFP-positive cells had, in fact, colonized into scales and fin rays and differentiated into bone-forming cells judged by position and cell shapes ( n =31/347, 3/278, 12/309, 6/105, for scales, dorsal, anal and caudal fins, respectively; number of fish with GFP-positive cells in scales and fin rays/number of embryos with GFP-positive somite cells at 12 h after irradiation) ( Fig. 4c ). For technical reasons, not all the irradiated embryos were individually followed, but we succeeded in retrospectively tracing labelled cells in scales and anal fins back to the ones originally observed in embryos ( n =13/187 for scales and 3/130 for anal fins; Fig. 4b–i ). Probably because of a smaller population of precursor cells for dorsal and caudal fin rays in somites, the labelling frequency of these fins were quite low under our experimental conditions. 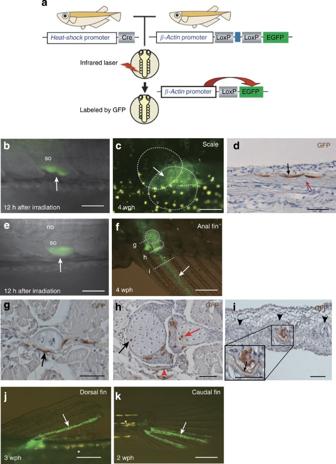Figure 4: Somite origin of scales and median fin rays is confirmed by IR-LEGO labelling. (a) IR-LEGO system. (b,e) Labelled somite cells (arrows) at 12 h after exposure to infrared laser. Dorsal views (c). Labelled cells inbcolonized on scales (arrow). Dotted circles show scales. (d) A histological section of the scale at the level shown as a dotted straight line inc. GFP-positive bone-forming cells (black arrow) are seen on the scale matrix (red arrow). (f) Labelled cells inecolonized on the anal fin ray (arrow) and its upper region including scales (dotted circles). (g–i) Histological sections at the levels shown inf. The arrow ingindicates bone-forming cells of the proximal radial. The black and red arrows inhindicate chondrocytes in the proximal and distal radials, respectively. The red arrowhead inhindicates bone-forming cells of the fin ray that are surrounding the proximal radial. The arrowheads inishow fin ray units. The arrow iniindicates bone-forming cells of the fin ray. (j,k) GFP-positive cells on dorsal and caudal fin rays, respectively.c,f,j,kare lateral views. Anterior to the left. GFP detection was performed by immunostaining ind,g–i. The asterisks show leucophores. no, notochord; so, somite. Scale bars, 50 μm (d,g–i), 100 μm (b,e), 500 μm (c,f,j,k). Figure 4: Somite origin of scales and median fin rays is confirmed by IR-LEGO labelling. ( a ) IR-LEGO system. ( b , e ) Labelled somite cells (arrows) at 12 h after exposure to infrared laser. Dorsal views ( c ). Labelled cells in b colonized on scales (arrow). Dotted circles show scales. ( d ) A histological section of the scale at the level shown as a dotted straight line in c . GFP-positive bone-forming cells (black arrow) are seen on the scale matrix (red arrow). ( f ) Labelled cells in e colonized on the anal fin ray (arrow) and its upper region including scales (dotted circles). ( g – i ) Histological sections at the levels shown in f . The arrow in g indicates bone-forming cells of the proximal radial. The black and red arrows in h indicate chondrocytes in the proximal and distal radials, respectively. The red arrowhead in h indicates bone-forming cells of the fin ray that are surrounding the proximal radial. The arrowheads in i show fin ray units. The arrow in i indicates bone-forming cells of the fin ray. ( j , k ) GFP-positive cells on dorsal and caudal fin rays, respectively. c , f , j , k are lateral views. Anterior to the left. GFP detection was performed by immunostaining in d , g – i . The asterisks show leucophores. no, notochord; so, somite. Scale bars, 50 μm ( d , g – i ), 100 μm ( b , e ), 500 μm ( c , f , j , k ). Full size image Interestingly, in most cases, GFP-positive fin rays were accompanied by GFP-positive radials (endoskeleton) ( Fig. 4f–i , Supplementary Fig. S5 ). This suggests that the fin rays and radials share a precursor cell population, although we cannot exclude the possibility that they are formed from multiple progenitor cell populations. Taken together, we confirmed the results of somite transplantation that bone-forming cells of scales and median fin rays are derived from the somite. Pectoral fin rays are derived from the LPM Additionally, we addressed the question of the embryonic origin of paired fin rays. Fish paired fins are homologous to tetrapod limbs. While limbs have only endoskeletal elements, paired fins have distal exoskeletal elements, fin rays, in addition to the proximal endoskeleton [29] . Like median fins, fin rays of paired fins have long been assumed to be neural crest in origin. To test this, we dissected dorsal neural tubes at the post-otic levels from double transgenic embryos ( β-actin-DsRed / osterix-EGFP ) at the 12-somite stage, and transplanted them into host embryos at the same AP levels. A population of neural-crest cells from the level of the anterior-most three somites was found to migrate into pectoral fin folds ( Fig. 5a left). However, none of these neural crest cells expressed GFP, suggesting that they did not contribute to fin rays ( n =0/11, Fig. 5b , right). We then examined the contribution of somites. We sequentially replaced each of the anterior-most three somites with a transgenic one and observed that cells from the second somite migrated into paired fins. However, they only differentiated into blood vessels in the fin fold, judged by position and morphology ( Fig. 5c , left), and again failed to express GFP ( n =0/8, Fig. 5d , right). We finally suspected the lateral plate mesoderm (LPM), which is known to contribute mesenchymal cells to the limb in amniotes. As the medaka LPM is too thin to be transplanted, we only conducted an IR-LEGO labelling experiment ( Fig. 5e ). A small number of LPM cells on the yolk sac lateral to the second somite were labelled by persistent GFP expression ( Fig. 5g ). Three weeks later, GFP-positive cells populated the fin rays of pectoral fins mostly together with radials ( n =10/15; number of fish with GFP-positive fin rays/number of embryos having GFP-positive fin buds) ( Fig. 5h ), and these cells indeed attached to the bone matrix, suggesting that LPM-derived cells contributed to pectoral fin rays ( Fig. 5i ). Further support was obtained by DiI-labelling of LPM cells in zebrafish embryos, demonstrating that they invade the pectoral fin folds where fin rays develop ( Fig. 6 ). Taken together, we conclude that bone-forming cells of pectoral fin rays are derived from the LPM. 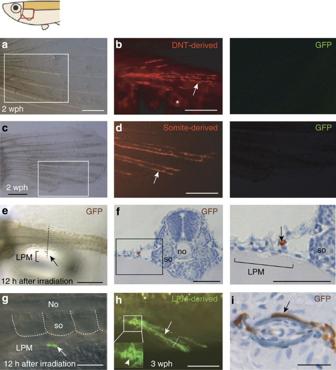Figure 5: LPM origin of pectoral fin rays. (a,b) Dorsal neural tubes (DNT) at the second somite level were removed from the Tg (β-actin-DsRed/osterix-EGFP) embryos at the 12-somite stage and transplanted into the wild-type host. (b) Left: DNT-derived DsRed-positive cells are found in the pectoral fin region shown as the box ina, but they are likely to be pigment cells or neurons judged from position and morphology. Right: no GFP-positive cells were found in the region shown inb(left). (c,d) Third somites were removed from the Tg at the 12-somite stage and transplanted into the wild-type host. (d) Left: somite-derived DsRed-positive cells are found in the pectoral fin region shown as the box inc, but they are likely to be blood vessels judged from position and morphology. Right: no GFP-positive cells were found in the region shown ind(left). (e,f) An example of GFP-positive LPM cells (arrows) 12 h after exposure to infrared laser. (f) The histological section at the level shown as the dotted line ine. Right: the enlarged picture of the region shown as the box in the left. The arrow indicates a LPM cell judged from position and morphology. (g) GFP-positive labelled cells in the LPM region. (h) Labelled cells distributed along the pectoral fin rays (arrow). The arrowhead shows endoskeletal fin radials. (i) The histological section at the level indicated as the dotted line inh. The arrow indicates GFP-positive bone-forming cells. Lateral views (a–d,h). Dorsal views (e,g). Pectoral fins ina,c,d, had been isolated, while those inb,hhad not been isolated. GFP detection ine,f,iwas performed by immunostaining. Asterisks indicate leucophores. no, notochord; so, somite. Scale bars, 50 μm (i), 100 μm (f,g), 200 μm (a–e), 500 μm (h). Figure 5: LPM origin of pectoral fin rays. ( a , b ) Dorsal neural tubes (DNT) at the second somite level were removed from the Tg ( β-actin-DsRed / osterix-EGFP ) embryos at the 12-somite stage and transplanted into the wild-type host. ( b ) Left: DNT-derived DsRed-positive cells are found in the pectoral fin region shown as the box in a , but they are likely to be pigment cells or neurons judged from position and morphology. Right: no GFP-positive cells were found in the region shown in b (left). ( c , d ) Third somites were removed from the Tg at the 12-somite stage and transplanted into the wild-type host. ( d ) Left: somite-derived DsRed-positive cells are found in the pectoral fin region shown as the box in c , but they are likely to be blood vessels judged from position and morphology. Right: no GFP-positive cells were found in the region shown in d (left). ( e , f ) An example of GFP-positive LPM cells (arrows) 12 h after exposure to infrared laser. ( f ) The histological section at the level shown as the dotted line in e . Right: the enlarged picture of the region shown as the box in the left. The arrow indicates a LPM cell judged from position and morphology. ( g ) GFP-positive labelled cells in the LPM region. ( h ) Labelled cells distributed along the pectoral fin rays (arrow). The arrowhead shows endoskeletal fin radials. ( i ) The histological section at the level indicated as the dotted line in h . The arrow indicates GFP-positive bone-forming cells. Lateral views ( a – d , h ). Dorsal views ( e , g ). Pectoral fins in a , c , d , had been isolated, while those in b , h had not been isolated. GFP detection in e , f , i was performed by immunostaining. Asterisks indicate leucophores. no, notochord; so, somite. Scale bars, 50 μm ( i ), 100 μm ( f , g ), 200 μm ( a – e ), 500 μm ( h ). 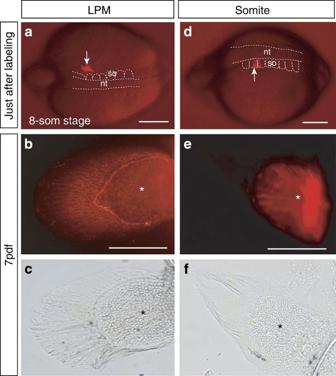Figure 6: DiI-labelled LPM cells contribute to the pectoral fin mesenchyme in zebrafish. (a,d) DiI was injected into the LPM and somite, respectively. (b,e) Pectoral fins of the embryos whose LPM had been injected with DiI exhibited labelled mesenchyme in their fin fold, whereas those whose somite had been injected with DiI did not exhibit labelled mesenchyme. The latter appeared to have labelled muscle in the endoskeletal part of the pectoral fin (this region is marked by asterisks). (c,f) Bright-field images of the panelsb,e, respectively. nt, neural tube; so, somite. Scale bars, 200 μm. Full size image Figure 6: DiI-labelled LPM cells contribute to the pectoral fin mesenchyme in zebrafish. ( a , d ) DiI was injected into the LPM and somite, respectively. ( b , e ) Pectoral fins of the embryos whose LPM had been injected with DiI exhibited labelled mesenchyme in their fin fold, whereas those whose somite had been injected with DiI did not exhibit labelled mesenchyme. The latter appeared to have labelled muscle in the endoskeletal part of the pectoral fin (this region is marked by asterisks). ( c , f ) Bright-field images of the panels b , e , respectively. nt, neural tube; so, somite. Scale bars, 200 μm. Full size image A previous study of somite transplantation in zebrafish using muscle-specific reporter lines ( alpha-actin promoter) revealed that muscle was derived from the transplant in pelvic fins [20] . The present study has extended the lineage analysis of the trunk mesoderm to specifically examine its contribution to the skeletal elements using the odontoblast/osteoblast-reporter medaka and IR-LEGO technique. The embryonic origin of vertebrate cranial skeleton (mesoderm and neural crest), as well as trunk endoskeletal elements such as vertebra (mesoderm) has been well studied in tetrapods [6] , [7] , [8] , [9] , [10] , [11] , [14] . In contrast, the origin of trunk exoskeleton was still enigmatic. The fish trunk neural crest was previously expected to produce ectomesenchyme and form skeletal derivatives [17] , [18] , but our results suggest that the trunk neural crest has no skeletogenic capability in teleosts, instead highlighting the dominant role of the mesoderm in the trunk exoskeleton. This further implies that the skeletogenic fate of the neural crest has been predominant in the cephalic region from the early stage of vertebrate evolution. Our results also provide new insights into the fish-to-tetrapod evolution. The evolution of scale is thought to be complex and we are unable to extrapolate our findings simply to what could have happened in vertebrate evolution [30] , [31] . However, if we follow the recently proposed idea that teleost elasmoid scales are odontogenic tissues [12] , [13] , the skeletogeneic fate of the somite-derived cells could have been realized in the trunk surface in ancestral fish. This ability could then become suppressed (or latent) during terrestrial evolution. The mechanisms underlying skeletogenic fate suppression remain unknown, but it could be achieved through inhibitory signals from the surrounding surface tissues. Altering genetic regulation of inhibitory signalling cascades might explain a phenomenon that some tetrapods develop integumentary skeletons in the dermis such as dermal scales in gymnophionans (amphibian); although their developmental origin remains elusive [4] . During the transition from fin to limb, exoskeletal elements (fin rays) in the distal part of paired fins disappeared, followed by the formation of distally expanded endoskeletal elements (digits) from the LPM-derived cell population [32] , [33] . The former changes have been mainly explained by the suppression (or latency) in the skeletogenic fates of the neural crest, because fin rays are thought to be of neural crest origin [3] , [34] . However, our study demonstrates that the digits and fin rays share the same developmental origin, LPM, implying that LPM mesenchymal cells are responsible for the loss of fin rays. Indeed, in most cases of our lineage analyses, both fin rays and radials were continuously labelled, suggesting that the LPM-derived mesenchyme forms both endoskeletal and exoskeletal components, depending on their locations. The formation of exoskeletons could depend on actinotrichia collagens secreted from the epidermis [35] . The ability of mesodermal cells to contribute to dermal bones has recently been recognized in the skull vault and the clavicle of the shoulder in chick and mouse [9] , [11] , [36] . Moreover, histogenic patterns of skeletogenesis (endochondral versus membranous) have been proposed to depend on the embryonic environments, rather than being intrinsic to cell lineages [37] . Our observations are consistent with these findings and confirm that neither the histogenic pattern nor the anatomical topology (exo- versus endoskeletons) is coupled with the developmental cell lineages. It is, therefore, possible that developmental pathways associated with skeletogenesis are shared between neural crest-derived and mesoderm-derived mesenchyme, upon which the anatomical pattern of vertebrate body may have attained the endless diversity we see today. Finally, our study implies that the earliest exoskeleton (dermal armors) was of a mixed composition, with both neural crest and mesodermal components. Recently, amphioxus was found to have Pax3/7-positive satellite-like cells, suggesting that they have already acquired an evolutionary precursor of somite-derived dermomyotome, a tissue that produces dermis [38] . In fact, they exhibit ‘lateral somitic wall cells (dermomyotome-like cells)’ adjacent to the epidermis [39] . Genetic machinery to create the trunk exoskeleton was probably elaborated in these dermomyotome-like cells and later co-opted by the cranial neural crest, or it was first assembled in the cranial neural crest and then co-opted by the trunk mesoderm. Alternatively, it may be most plausible that mesenchymal cell populations, regardless of developmental origins, acquired skeletogenic ability, possibly throughout the entire body, at an early stage of vertebrate evolution. However, our knowledge is still limited to the teleost, the most modern fish, and further evolutionary insights should await similar lineage analyses in vertebrates whose ancestors diverged earlier, such as sharks. Tissue transplantation Double transgenic fish used as donors were obtained by across between Tg ( beta-actin-DsRed ) [40] and Tg ( osterix-EGFP ) [41] . Tissue transplantation was performed essentially according to previous zebrafish experiments [19] , [20] , with some modifications. Both donor and host embryos were dechorionated with hatching enzyme. After the head and yolk were removed, the trunk regions of donor embryos were treated with 20 mg ml −1 pancreatin (Wako) for several minutes at room temperature. Dorsal neural tubes were then dissected and cut into single- or two-somite in width by a long fine-drawn glass needle and kept in 10% FBS. Single or two successive somites were also prepared in the same way. Wild-type (d-rR or T5 strain) host embryos were mounted in 1% low-melting temperature agarose in a plastic petri dish (3.5 cm in diameter). Neural tubes or somites of host embryos were extirpated at the same regions as donor tissues with a glass needle, and the donor tissues were transplanted into the extirpated space by another glass needle with a round tip. The transplanted embryos were incubated at 28 °C to the hatching stage. Tissues and embryos were always kept in Yamamoto’s Ringer solution [42] containing 200 U penicillin per ml and 200 mg ml −1 streptomycin. IR-LEGO operation Construction of the transgene β-actin -loxP[ DsRed ]- EGFP was as follows: a cassette consisting of 3.7 kb of medaka β-actin promoter, lox P, part of DsRed2 gene (nonsense gene), lox P and EGFP gene was inserted into the EcoRI/NotI site of pDsRed2-1 (Clontech). While Tg ( hsp - cre ) [28] were homozygous, Tg ( β-actin -loxP[ DsRed ]- EGFP ) were in the heterozygous state because homozygous fish are very weak and unhealthy. Embryos to be irradiated were obtained by a cross between Tg ( hsp - cre ) and Tg ( β-actin -loxP[ DsRed ]- EGFP ). They were embedded in 2% methylcellulose solution/Yamamoto’s Ringer for stable positioning of the targets on glass base dishes (Matsunami 0.08–0.12 mm thickness, code D110400). The caudal most somites or LPM were irradiated with infrared laser (16–18 mW for one second, × 40 objective) using IR-LEGO microscope system (Sigma Koki IR-LEGO-1000) [23] , [24] . To confirm successful labelling, we checked GFP expression in the target region at 12 h after IR irradiation. The GFP-expressing cells maintained fluorescence throughout life, as their transgene has recombined by the Cre recombinase locally induced with heat-shock. Whole-mount in situ hybridization Embryos were fixed with 4% paraformaldehyde/PBS overnight at room temperature. Hybridization was performed with DIG-labelled RNA probes at 65 °C overnight. Signals were detected by alkaline-phosphate-conjugated anti-DIG Fab fragments (1:8,000) (Boehringer Mannheim). Neural tubes were embedded in 1% low-melting temperature agarose during the whole process. The primers for foxd3 probes were 5′-GATGACTTGGAAGATGAAATCG-3′, 5′-ACACCCCGATGATGTTTTCTATAC-3′. The same method was applied for in situ hybridization of neural tubes except that samples were fixed for 2 h and that they were embedded in 1% low-melting temperature agarose throughout the process. Histological analysis The trunk region including fins was dissected and fixed with 4% paraformaldehyde/PBS overnight at room temperature, followed by whole-mount immunostaining. The primary antibodies (anti-GFP, Medical & Biological Laboratories or Clontech (JL-8))(anti-DsRed, Clontech #632496) and secondary antibody (biotin-conjugated anti-rabbit IgG (Sigma)) were used at a 1:250 dilution. Staining was done using VECTASTAIN Elite ABC kit, VECTOR. The specimens were embedded in a Technovit 8100 (Heraeus Kulzer, Wehrheim) and sectioned at a 5-μm thickness. In the experiment that detects infrared laser-induced GFP expression in fin skeleton, immunostaining was performed on the histological sections made from paraffin-embedded specimens. How to cite this article: Shimada A. et al . Trunk exoskeleton in teleosts is mesodermal in origin. Nat. Commun. 4:1639 doi: 10.1038/ncomms2643 (2012).